A digital laser for on-demand laser modes Customizing the output beam shape from a laser invariably involves specialized optical elements in the form of apertures, diffractive optics and free-form mirrors. Such optics require considerable design and fabrication effort and suffer from the further disadvantage of being immutably connected to the selection of a particular spatial mode. Here we overcome these limitations with the first digital laser comprising an electrically addressed reflective phase-only spatial light modulator as an intra-cavity digitally addressed holographic mirror. The phase and amplitude of the holographic mirror may be controlled simply by writing a computer-generated hologram in the form of a grey-scale image to the device, for on-demand laser modes. We show that we can digitally control the laser modes with ease, and demonstrate real-time switching between spatial modes in an otherwise standard solid-state laser resonator. Our work opens new possibilities for the customizing of laser modes at source. Laser beam-shaping tools [1] have matured over the past few decades to allow external (to the laser cavity) reshaping of a laser beam to a desired transverse profile, and may be implemented by a variety of methods, for example, by diffractive optical elements, free-form optics or more recently by digital holograms written to a spatial light modulator (SLM). However, there are advantages to rather shaping the light inside the laser cavity (intra-cavity laser beam shaping) and this has been a subject of interest for a number of years [2] , [3] , [4] , with several design techniques available [5] , [6] , [7] , [8] , [9] , [10] , some of which have successfully been implemented, for example, using phase-only [11] , [12] , [13] , [14] , amplitude-only [15] , [16] and phase–amplitude combination [17] optical elements for spatial mode selection. All of these techniques require custom optics and in some cases (for example, Bourderionnet. et al. [17] ) additional external beam-shaping optics, a wavefront sensor and an optimization routine to iterate towards the desired phase profile. There have also been attempts at dynamic intra-cavity beam control with deformable mirrors [18] , [19] , [20] , [21] , [22] , [23] , but such elements have very limited stroke, are limited in the phase profiles that can be accommodated [18] , [19] , and thus have found little application in laser mode shaping. Rather, such mirrors have been instrumental in high-power applications such as correcting mode distortions (for example, because of thermal load) or in maximizing energy extraction and optimization of laser brightness [20] , [21] , [22] , [23] . To date, no technique has been demonstrated for on-demand selection of arbitrary laser modes in real-time. Here we overcome the aforementioned limitations through the use of intra-cavity digital holograms, implemented on a phase-only reflective SLM, to form a rewritable holographic mirror in place of the standard laser cavity mirror, the digital laser. This allows an on-demand mode selection with high resolution and with a very wide dynamic range of phase values. This approach simplifies significantly the task of intra-cavity beam shaping, reduces the time to test concepts and only supposes the ability to create appropriate grey-scale images. To put this another way, creating custom modes is reduced to that of creating pictures of what you want, and the tools to do this are very well established (see, for example, the vast literature on shaping light with digital holograms). The advantage of our approach over that of others is that the abovementioned capability comes at minimal complexity: one only requires a commercial SLM and an otherwise standard laser cavity. Moreover, all the known tools for intra-cavity mode selection may be implemented in the digital laser. We demonstrate that the digital laser can mimic a conventional stable cavity and verify on-demand mode selection by dynamically changing the mirror hologram to output a variety of laser modes in real-time. We accomplish this feat by ‘playing a video’ inside a laser cavity, requiring a shift in our thinking of mode control in laser resonators. Realizing a digital laser Our laser cavity, as shown in Fig. 1 , consists of a conventional folded resonator configuration with an Nd:YAG laser crystal as the gain medium (see Methods section). What is unconventional is the use of a phase-only reflective SLM as the back optical element of the cavity. The SLM is used to display computer-generated holograms, sometimes called digital holograms, encoded as pixelated grey-scale images. The SLM is calibrated such that a full phase cycle from 0 through 2 π is represented graphically by grey-scale colours ranging from white through black, in 256 levels (8-bit encoding). For example, a linear ramp in colour from white to black would represent a linear ramp in phase from 0 to 2 π , otherwise known as a diffraction grating. In a similar way, virtually any desired phase may be encoded using the SLM. One can consider the colour change on the SLM as equivalent to the depth change in a standard diffractive optical element, and herein lies the advantage: it is easy to change colours in images but rather time consuming to refabricate depth changes in diffractive optical elements. As the device acts as our back mirror and displays a digital hologram to change the phase of the reflected light, we will refer to it as a digitally addressed holographic mirror (or holographic mirror for short). The key properties required of the SLM for this application are high resolution, high efficiency, high reflectivity at the desired polarization, small phase–amplitude crosstalk, reasonable damage threshold and a large phase shift at the laser wavelength. 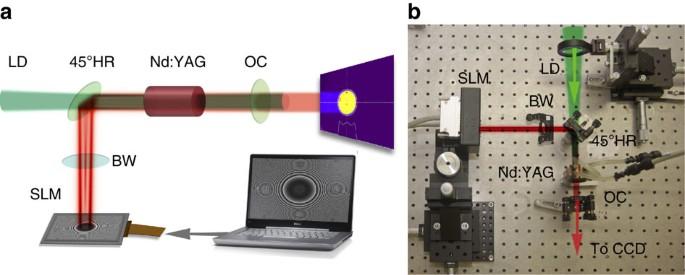Figure 1: Concept and experimental realization of the digital laser. (a) Schematic of the digital laser concept showing the SLM, Brewster window (BW), high reflectivity (HR) mirror at an angle of 45°, Nd:YAG gain medium pumped by an external laser diode (LD) source and the output coupler (OC). (b) Photograph of the experimental set-up. Figure 1: Concept and experimental realization of the digital laser. ( a ) Schematic of the digital laser concept showing the SLM, Brewster window (BW), high reflectivity (HR) mirror at an angle of 45°, Nd:YAG gain medium pumped by an external laser diode (LD) source and the output coupler (OC). ( b ) Photograph of the experimental set-up. Full size image The laser was optically pumped by a high-power laser diode that was coupled into the cavity through a mirror coated for high transmission at the diode wavelength (808 nm) and high reflectance at the lasing wavelength (1064, nm). This folding mirror forms an L-shaped cavity so that the high-power diode beam does not interact with the SLM, thus avoiding damage. An important feature of the cavity is the intra-cavity Brewster window to force the laser to oscillate in the desired polarization for the SLM (vertical in our set-up). The light is passed out of the cavity through the output coupler (OC). As a proof-of-principle experiment, we programmed the holographic mirror to mimic a conventional concave mirror with a radius of curvature, R , chosen to ensure that the resonator formed a stable plano-concave cavity ( Fig. 2a ). This requires a digital hologram of a lens to be programmed to the SLM, with focal length f=R , so that the hologram mimics the curvature of the mirror. 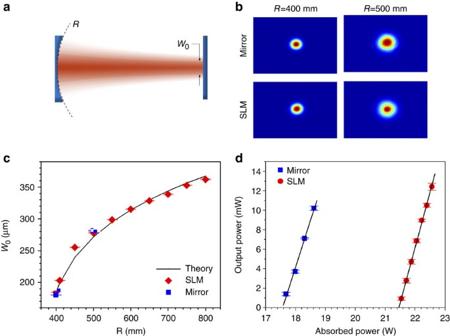Figure 2: Comparison of the digital laser to an equivalent plano-concave laser. (a) Schematic of the stable plano-concave resonator with a waist plane at the flat OC. (b) Measured intensity profiles for two curvature cases (R=400 and 500 mm), comparing the digital laser output (SLM) with that of physical mirrors (Mirror). (c) The change in measured beam size with digitally imposed curvature matches the theoretical curve. (d) The threshold of the digital laser is higher than that of the conventional laser owing to the additional losses from the SLM shown here for theR=400 mm case. The black lines are fits to the data and error bars are s.d.. The waist size (at the flat OC) of the Gaussian mode that oscillates in such a cavity may be described analytically as [2] : Figure 2: Comparison of the digital laser to an equivalent plano-concave laser. ( a ) Schematic of the stable plano-concave resonator with a waist plane at the flat OC. ( b ) Measured intensity profiles for two curvature cases ( R =400 and 500 mm), comparing the digital laser output (SLM) with that of physical mirrors (Mirror). ( c ) The change in measured beam size with digitally imposed curvature matches the theoretical curve. ( d ) The threshold of the digital laser is higher than that of the conventional laser owing to the additional losses from the SLM shown here for the R =400 mm case. The black lines are fits to the data and error bars are s.d.. Full size image where L is the effective length of the resonator and λ is the laser wavelength. Before testing the digital laser, two physical concave mirrors were used (separately) in the same set-up in place of the SLM, and the Gaussian beam size was recorded at the output. The results for these two cases, R =400 and 500 mm, are shown in Fig. 2b and plotted in Fig. 2c together with the theoretical curve, following equation (1). The same test curvature examples were programmed digitally and are shown alongside the physical mirror measurements in Fig. 2b . From a mode selection perspective, the laser performs identically in the two configurations. Next, as the digital hologram’s programmed curvature was changed ( Fig. 2c ) the measured output Gaussian beam size changed in accordance with equation (1). This confirms that the digital laser behaves as a standard stable cavity and it is clear from the results that the SLM mimics the stable cavity with high fidelity. In addition to confirming the desired behaviour of the digital laser, this experiment also brings to the fore another practical advantage: whereas with physical mirrors it is commonplace to have a limited and discrete selection on hand, with the digital approach virtually any mirror curvature can be created, on demand, by simply changing the grey-scale image representing the digital hologram, and is limited only by the resolution of the SLM used. The higher losses of the SLM do manifest themselves as a higher threshold for lasing, as noted in Fig. 2d . The losses are due to the overall diffraction efficiency of the device as well as the losses due to the fill factor. These two factors can reduce the apparent reflectivity of the SLM mirror by 15–20%. On-demand laser modes Next, we employ the digital laser to select the well-known Hermite–Gaussian, Laguerre–Gaussian, super-Gaussian (flat-top) and Airy beams. The digital laser may be used to implement amplitude-only, phase-only or amplitude and phase modulation by simply altering the digital hologram (grey-scale picture) written to the device. The SLM is a phase-only device, yet many of the desired holograms require both amplitude and phase change to the field. To achieve this, we make use of the well-known method of complex amplitude modulation [24] , [25] , [26] , because this is suitable for implementation on SLMs. There are several means by which to implement this (see Arrizon et al. [25] , [26] and references therein), and for the benefit of the reader we briefly outline one approach used in the creation of our modes. Consider for example a desired field u ( x , y )= u 0 exp( i φ), with u 0 the real amplitude and φ the phase of the desired beam. To encode the amplitude term, we introduce high spatial frequency modulation in the form of a checkerboard pattern with alternating phases between two values. The two phases are chosen so that their average value is equal to the desired complex value. For example, if the two phase values are given by A =exp( i φ+ i α) and B =exp( i φ– i α), then the desired amplitude u 0 may be expressed as u 0 =cos α . This checkerboard may be varied spatially to create arbitrary amplitude modulation as a function of position. A graphical interpretation of the process is shown in Fig. 3a , where the modulation between two phase-only values ( A and B ) gives an average return of C , which is no longer on the unit circle in the complex plane, that is, amplitude modulation of the input field. The checkerboard corresponding to this is shown in Fig. 3b . This can be understood from basic diffraction theory: some of the incoming light is diffracted by the checkerboard grating into higher diffraction orders, so that the resulting light in the desired order is now less than before. In this sense the desired light has been amplitude modulated, although the pattern on the SLM is phase-only. 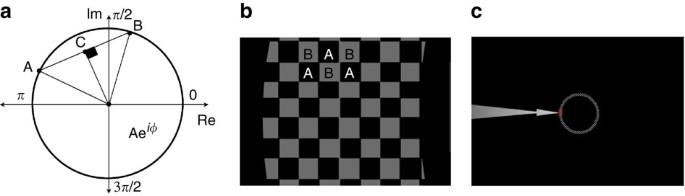Figure 3: Complex amplitude modulation concept. (a) Schematic of the complex plane showing two phase-only values,AandB, lies on the unit circle (unit amplitude). The average of these is vectorC, representing amplitude modulation as it is not on the unit circle. (b) Example of a checkerboard pattern of the two phase valuesAandB. (c) Zoomed out image ofbshowing the complete annular ring created with this checkerboard pattern to result in zero transmission in the annular ring. Figure 3: Complex amplitude modulation concept. ( a ) Schematic of the complex plane showing two phase-only values, A and B , lies on the unit circle (unit amplitude). The average of these is vector C , representing amplitude modulation as it is not on the unit circle. ( b ) Example of a checkerboard pattern of the two phase values A and B . ( c ) Zoomed out image of b showing the complete annular ring created with this checkerboard pattern to result in zero transmission in the annular ring. Full size image Thus, although our SLM is calibrated for a phase-only response from 0 (black) to 2 π (white), appropriate holograms can result in amplitude variations from 0 to 1. An example of a high-loss annular ring is shown in Fig. 3c , with the zoomed-in checkerboard shown in Fig. 3b . The selection of the Hermite–Gaussian and Laguerre–Gaussian modes ( Fig. 4 ) exploited complex amplitude modulation to implement amplitude modulation on the phase-only SLM [24] , [25] , [26] . In other words, the SLM can be used to create customized apertures, for example, the fine wires (loss-lines) used in the past for Hermite–Gaussian mode selection [2] , [3] . The digital hologram for the creation of the radial Laguerre–Gaussian beam ( p =1, l =0) comprised a high-loss annular aperture, together with a phase-only radius of curvature. In this case, the checkerboard consisted of the two phase values, 0 and π , for a resultant of zero amplitude inside an annular ring. This low-loss ring was positioned at the zero of the first radial Laguerre–Gaussian function to select the pure LG 10 mode shown in Fig. 4 . The radius of curvature was used to select and control the mode size, following equation (1). Many techniques exist for the design of intra-cavity diffractive optics [5] , [6] , [7] , [8] , [9] , [10] for particular mode selection, all of which may readily be applied to the digital laser. We illustrate this in Fig. 4 where an Airy beam [27] and flat-top beam [7] are created by phase-only digital holograms. 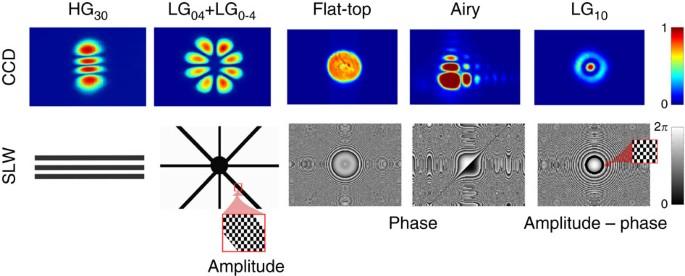Figure 4: Customized spatial modes by amplitude and phase modulation. By complex amplitude modulation, a customized set of high-loss regions create a Hermite–Gaussian beam (n=3,m=0) and a superposition of Laguerre–Gaussian beams (p=0,l=±4) as the laser output. By phase-only modulation, a flat-top beam and Airy beam are created as the stable modes of the cavity. Combining amplitude and phase effects allows for the selection of a Laguerre–Gaussian beam (p=1,l=0) of a chosen size. Figure 4: Customized spatial modes by amplitude and phase modulation. By complex amplitude modulation, a customized set of high-loss regions create a Hermite–Gaussian beam ( n =3, m =0) and a superposition of Laguerre–Gaussian beams ( p =0, l =±4) as the laser output. By phase-only modulation, a flat-top beam and Airy beam are created as the stable modes of the cavity. Combining amplitude and phase effects allows for the selection of a Laguerre–Gaussian beam ( p =1, l =0) of a chosen size. Full size image Finally, we note that the switching from one mode to another required nothing more than a change to the grey-scale image making up the digital hologram—no realignment and no additional optical elements were necessary. Traditionally, to create the spectrum of modes shown in Fig. 4 would require several laser resonator set-ups, each with a custom (expensive) optic. We exploit the versatility of the digital laser by operating the laser in ‘video’ mode: the fundamental mode of the laser was changed in real-time (at video fresh rates) by dynamically changing the digital hologram. The results are shown in Supplementary Movies 1 and 2 , the first time this has ever been done in a laser and represent a shift in thinking about laser resonators. To illustrate this technique’s applicability for intra-cavity mode control with the digital laser, we consider the generation of high-order modes and their superpositions in the laser cavity using complex amplitude modulation. In Fig. 5 , we illustrate higher-order modes from the Laguerre–Gaussian basis, and in Fig. 6 we show a very high superposition state of the Laguerre–Gaussian modes with azimuthal indices of l =25 and −25, creating a petal-like structure with 50 lobes. This is the highest pure azimuthal combination created in a laser that we are aware of. It is clear from these examples that a myriad of modes may be created within the laser cavity using our approach. 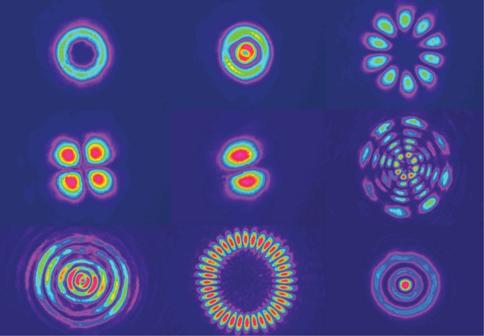Figure 5: Higher-order Laguerre–Gaussian modes. An example range of modes created with the digital laser. Figure 5: Higher-order Laguerre–Gaussian modes. An example range of modes created with the digital laser. 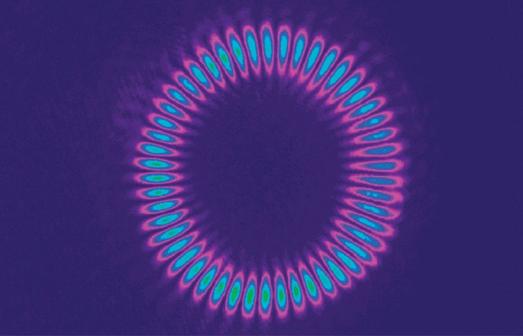Figure 6: A superposition of two high-order azimuthal modes. Two Laguerre–Gaussian modes of opposite but equal azimuthal index, and of azimuthal order |l|=25, are combined coherently in the digital laser to produce this high-order superposition. Full size image Figure 6: A superposition of two high-order azimuthal modes. Two Laguerre–Gaussian modes of opposite but equal azimuthal index, and of azimuthal order | l |=25, are combined coherently in the digital laser to produce this high-order superposition. Full size image All the beam shapes shown here were possible because the holograms fell well within the resolution of the SLM. At 800 × 600 pixels of pitch 20 μm, the resolution is significantly higher than that of an adaptive mirror but substantially lower than that of a typical diffractive optical element. As the number of pixels decreases for each phase ramp of 0–2 π , so does the diffraction efficiency, as well as the functionality of the hologram (for example, Moiré patterns will degrade the resulting beam). Nevertheless, for a wide range of typical beam shapes, the standard devices more than suffice; moreover, SLM resolution has tended to increase of late. We note from our results that two conditions must be simultaneously satisfied for the digital laser to function: the gain of the laser must be sufficiently high to overcome the losses, but the intra-cavity circulating intensity must not exceed the damage threshold of the SLM. We manage this by virtue of a high-power pump source and an L-shaped cavity, but there are several other valid approaches (for example, increasing the doping concentration of the crystal). When these conditions are balanced, the digital laser functions as designed. We also point out that all of the techniques we used in designing the holograms for mode selection are standard and well known, that is, no new tools are needed to implement the digital laser approach. We have illustrated this point by creating modes traditionally generated by phase-only diffractive optical elements (for example, Airy beam), amplitude-only filters (for example, Hermite–Gaussian beams) and combinations of the two (high-order Laguerre–Gaussian beams). Importantly, all the modes that we have shown here required only a change to a picture—no new optics and no additional alignment of the laser cavity. It is the simplicity of our approach that makes it so powerful: we offer a direct and easy means to mode control, suitable with standard tools, without any special optics and only a commercial SLM, which we can assume many researchers are familiar with and have access to. This makes our approach accessible to all. In conclusion, we have demonstrated a novel digital laser that allows arbitrary intra-cavity laser beam shaping to be executed on the fly. This differs substantially from other intra-cavity laser beam-shaping approaches as only a grey-scale image needs change for the laser mode to be selected. We have shown that the digital laser can replicate conventional stable resonator cavities as well as ‘custom’ laser resonators to produce more exotic laser modes. The digital laser is at present limited in the power that it can output, but this may be overcome with careful engineering of bespoke liquid crystals. Just as SLMs external to the laser cavity have proved an excellent means for testing high-power beam-shaping elements before fabrication, and have in the process opened up many avenues for low-average-power applications of structured light (for example, holographic optical tweezers), the digital laser may well become an robust, easy-to-implement, test bed for intra-cavity beam-shaping ideas. Moreover, as the digital laser is rewritable it allows for dynamic intra-cavity beam shaping, as we have shown by ‘playing a video’ inside a laser for the first time. Applications of this would range from controlling thermal lensing and aberrations in real-time to real-time mode control and switching. Customized laser modes are now only a picture away. Laser cavity and SLM Several SLMs were used in the testing of the digital laser, and finally a Hamamatsu (LCOS-SLM X110468E) series device was selected for the digital laser. Previous tests with other SLMs failed mainly because of the phase–amplitude coupling that becomes pronounced during intra-cavity operation. The gain medium was a 1% doped Nd:YAG crystal rod with dimension of 30 mm (length) by 4 mm (diameter). The crystal was end-pumped with a 75-W Jenoptik (JOLD 75 CPXF 2P W) multimode fibre-coupled laser diode operating at 808 nm. The OC (flat curvature) had a reflectivity of 60%, whereas the SLM had a measured reflectivity of 91% at the desired polarization (vertical) and 93% at the undesired polarization (horizontal). To force the cavity to lase on the vertical polarization, an intra-cavity Brewster plate was used. On this polarization, calibration tests on the SLM reveal typical efficiencies of ~86% into the first order and ~1% into the zeroth order. In the intra-cavity configuration, this large difference results in suppression of the zeroth order because of the significantly higher round trip losses, and thus the SLM could be operated at normal incidence and without a grating. The SLM efficiency had a s.d. of ~0.4% across all grey levels, that is, minimal amplitude effects during phase modulation. The nominal length of the cavity was ~390 mm but was determined to have an effective length of 373 mm to compensate for the small thermal lensing due to pump absorption in the crystal as well as the refractive index of the crystal. The effective length was used in all calculations for the mode sizes. The resonator output was 1:1 imaged onto a Spiricon CCD camera for intensity measurements, and could also be directed to a second SLM for modal decomposition studies. For far-field tests, the first lens of the telescope was removed. How to cite this article: Ngcobo, S. et al. A digital laser for on-demand laser modes. Nat. Commun. 4:2289 doi: 10.1038/ncomms3289 (2013).